Quantum metrology with parametric amplifier-based photon correlation interferometers Conventional interferometers usually utilize beam splitters for wave splitting and recombination. These interferometers are widely used for precision measurement. Their sensitivity for phase measurement is limited by the shot noise, which can be suppressed with squeezed states of light. Here we study a new type of interferometer in which the beam splitting and recombination elements are parametric amplifiers. We observe an improvement of 4.1±0.3 dB in signal-to-noise ratio compared with a conventional interferometer under the same operating condition, which is a 1.6-fold enhancement in rms phase measurement sensitivity beyond the shot noise limit. The improvement is due to signal enhancement. Combined with the squeezed state technique for shot noise suppression, this interferometer promises further improvement in sensitivity. Furthermore, because nonlinear processes are involved in this interferometer, we can couple a variety of different waves and form new types of hybrid interferometers, opening a door for many applications in metrology. Interferometers are such fundamental devices that they are the irreplaceable elements in precision measurement and have wide applications in modern metrology [1] . The state of the art is the laser interferometer for gravitational wave detection [2] . However, because of the vacuum quantum noise injected into the unused port, the sensitivity of the interferometers in precision phase measurement is limited to the shot noise limit (SNL): Δ φ SNL =1/ with N as the photon number sensing the phase change [3] , [4] . The SNL is also known sometimes as the standard quantum limit (SQL), which is set for interferometry with classical fields. It was pointed out by Caves [3] that the vacuum noise can be suppressed by using the squeezed state of light. Soon after, sub-SNL interferometry was demonstrated experimentally [5] , [6] . Recently, such a strategy was applied to the laser interferometers for gravitational wave detection in a prototype device [7] and in GEO600 (ref. 8 ). Following this approach, different types of quantum states [9] with special noise behaviour are studied for quantum noise suppression to improve the sensitivity of a conventional interferometer (CI). Quantum entanglement, which allows the correlation of quantum fluctuations of distinct systems, can also be used to subtract out quantum noise via quantum destructive interference [10] , [11] . Reducing noise is the most straightforward way to increase the sensitivity of an interferometer. On the other hand, the sensitivity of an interferometer can also be improved by signal enhancement. This is the approach in recent research using the so-called NOON state, a photon number maximally entangled state, for improving phase measurement sensitivity [12] , [13] , [14] . The NOON states produce an interference fringe with super resolution that is more sensitive to phase change than CIs [15] . The Heisenberg limit, with a phase measurement sensitivity of Δ φ HL =1/ N , can be reached with this strategy in principle. It was claimed and experimentally shown that the SQL can be beaten by a projected NOON state with post-selection detection [16] . However, a further analysis shows that challenges still exist for surpassing the SQL with post-selection [17] . NOON-state interferometry beyond four photons was also demonstrated [18] . However, difficulty in obtaining NOON states with larger photon numbers hinders the practical applications of such a scheme. CIs use beam splitters or the equivalent as the basic elements. A non-conventional approach for interferometry was adopted by Yurke et al. [19] , who, in the quest for the Heisenberg limit, proposed to use parametric processes for wave splitting and recombination to form a non-conventional SU(1,1) interferometer. A similar approach was used by Jacobson et al. [20] who used a cavity-QED device to split a coherent state into a Schrödinger cat-like superposition state. Ou [21] also proposed to use a hypothetical interaction to split an N-photon state into a NOON state. Such an interaction was later realized by Leibfried et al. [22] via a quantum simulator in a trapped ion system. This was the first realization of a non-conventional interferometer (NCI) even though the quantum number is small (3 at most). It should be noted that recently there is another class of interferometers that measures a ‘nonlinear’ phase shift [23] , [24] , [25] , [26] , which is induced in a nonlinear process. The phase measured there is totally different from the phase we measured here and has a sensitivity limit that follows different photon number scaling laws [24] , [25] , [26] . Moreover, the interferometrical technique used there is still the conventional one using beam splitters. In this Article, we report the experimental implementation of the SU(1,1) NCI with parametric amplifiers for precision phase measurement. However, different from the original proposal by Yurke et al. [19] , which also suffers the shortcomings of low photon number, we adopt a variation proposed by Plick et al. [27] to use coherent state injection for photon number ‘boost’. We initially reported its classical version [28] . Here we concentrate on the quantum nature of its performance. We find that the fringe size (that is, the peak-to-peak output intensity) of the interferometer is increased via parametric amplification while the noise level is kept low, close to vacuum noise level, due to destructive quantum interference. We compare the performance of our NCI with a conventional Mach–Zehnder (MZ) interferometer and observe an improvement of 4.1 dB in signal-to-noise ratio under the same phase-sensing intensity conditions. As a CI operates at the SNL, the phase measurement sensitivity of our NCI beats the SNL by a factor of 1.6 in root-mean-square value (rms). The enhancement is mostly limited by the losses inside the interferometer, but unlike the squeezed state scheme, our interferometer is less sensitive to the external losses such as detector inefficiency. Like the NOON-state scheme, the improvement in sensitivity in our approach here is because of the increase in the signal related to the phase change with an amplified fringe. However, our scheme is not limited by photon number. Comparison between different types of interferometers As mentioned before, the increase in phase measurement sensitivity in the NCI is not due to noise reduction but due to signal enhancement. In order to demonstrate this, we experimentally compare it with a CI, which works at the SNL. As the SNL is related to the phase-sensing photon number. We make the comparison under the same condition of phase-sensing light intensity. We first look at the principle of operation for the two kinds of interferometers. The schematic diagrams of an SU(1,1) NCI and a conventional MZ interferometer (CI) are shown in Fig. 1a,b . For the NCI, beam splitters are replaced by parametric amplifiers (PA1, PA2), which amplify the incoming ‘signal’ field and produce a correlated ‘idler’ field through nonlinear interaction. The ‘idler’ input field is labelled as and is in vacuum. In the present realization of NCI, the parametric amplifier is based on non-degenerate four-wave mixing in hot Rb-85 atomic vapour cells [29] (see Methods for the details of the experimental arrangement). A full quantum analysis of the NCI is presented in ref. 30. For completeness, we briefly present it here. 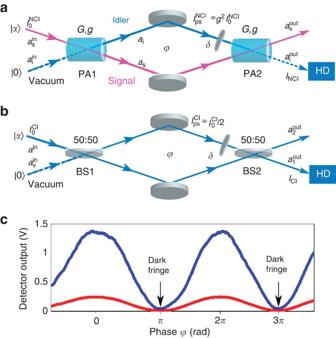Figure 1: Schematic diagram and interference fringes for two types of interferometers. (a) An SU(1,1) NCI; (b) a conventional MZ interferometer. PA, parametric amplifier;G,g, amplitude gains of PAs;φ, overall phase shift;δ, small phase change;I0, average input intensity;Ips, the intensity that senses the phase change; HD, homodyne detection. (c) The interference fringes at the outputs of the NCI (blue) and the CI (red) with the same phase-sensing intensity==60 μW. The fringe enhancement of NCI to CI isBS=5.5=7.4dB. The input–output relation for a parametric amplifier is given by: Figure 1: Schematic diagram and interference fringes for two types of interferometers. ( a ) An SU(1,1) NCI; ( b ) a conventional MZ interferometer. PA, parametric amplifier; G , g , amplitude gains of PAs; φ , overall phase shift; δ , small phase change; I 0 , average input intensity; I ps , the intensity that senses the phase change; HD, homodyne detection. ( c ) The interference fringes at the outputs of the NCI (blue) and the CI (red) with the same phase-sensing intensity = =60 μW. The fringe enhancement of NCI to CI is B S =5.5=7.4 dB . Full size image where G is the amplitude gain and g 2 = G 2 −1. With an overall phase shift φ in the idler arm, we obtain the output fields of the interferometer: with ( φ )= G 2 e − iφ + g 2 , ( φ )= Gg (1+ e − iφ ) as the phase-sensitive gains. For a coherent state | α injected in the signal input and vacuum in the idler input, we obtain the output intensity in the idler port or one of the outputs of the NCI as where ≡ g 2 ( +1) is the intensity of the phase-sensing field (idler field in Fig. 1a ) with ≡| α | 2 as the input intensity. For >>1, ≈ g 2 . A conventional MZ interferometer shown in Fig. 1b , on the other hand, has a fringe given by with 50:50 beam splitters and a coherent state |α input. ≡ /2=|α| 2 /2 is the phase-sensing intensity for the CI. Since the sensitivity of an interferometer is related to the photon number inside the interferometer, for a fair comparison between NCI and CI, we set = , which can be achieved by adjusting , independently. Therefore, we see from equations (3) and (4) that, under the condition of the same phase-sensing intensity, the output of the NCI is 2 G 2 times that of the CI. The increase in the signal for the NCI in Fig. 1a is not surprising because of the amplification within the interferometer. However, as is well known, for any amplifier, the amplification of signal is also accompanied by the amplification of the noise. So, the signal-to-noise ratio at best does not change in the process [31] . Fortunately, it is not the case for the NCI discussed here. From equation (2), at dark fringe when φ =(2 n +1) π , we have . However, since is in vacuum, the output of the NCI is at vacuum noise level, just like the CI at dark fringe. Thus, the signal in the NCI is increased while the noise level is not and we should expect an enhancement of 2 G 2 in signal-to-noise ratio of the NCI over the CI. What happens here for the NCI is that although each amplifier increases signal and noise together, the first parametric amplifier (PA1) produces two fields (two arms of the NCI) that are quantum mechanically entangled [32] , [33] , [34] so that their noises are also correlated, and a destructive interference occurs at the second parametric amplifier (PA2) when the interferometer is operated at dark fringe so that most of the amplified noise from PA1 are cancelled and only the vacuum noise is left [35] . Therefore, the NCI increases the signal while it keeps the noise unchanged, leading to an enhancement in signal-to-noise ratio for phase measurement as compared with the CI. Experimental results Figure 1c shows the interference fringes observed for both NCI and CI with the same phase-sensing intensity = . The fringe size of the NCI is bigger than that of the CI because of the amplification at PA2, which leads to an enhancement in the phase signal. This is the key difference between an NCI and a CI. When operated at dark fringe with a small phase change: φ =(2 n +1) π + δ ( δ <<1, n =integer), we obtain from equations (3) and (4) the change in the output intensities of the two interferometers due to δ as: So, the signal is enhanced by B S ≡Δ I NCI /Δ I CI =2 G 2 for the same δ and = . The fringe enhancement in Fig. 1c is B S =5.5=7.4 dB. The noise performance of the NCI is measured by homodyne detection (HD) method at the idler output port, as shown in Fig. 1a . The results are shown in Fig. 2 together with their graphic representation. The trace in dark blue in Fig. 2c shows the noise level at the output of the NCI when the phase is scanned. The minimum noise occurs at dark fringe when there is a destructive quantum interference at PA2. This is in contrast to the trace in yellow when one arm of the NCI is blocked and there is no interference effect. The trace in yellow corresponds to two uncorrelated amplifiers in series, as depicted in Fig. 2b . The traces in green and dark brown respectively show the noise levels for individual amplifiers when the other one is not active. Notice that at some phases, the output noise level (the trace in dark blue) of the NCI is even lower than the amplified noise levels of individual amplifiers (the traces in green and dark brown) as a result of noise cancelation. 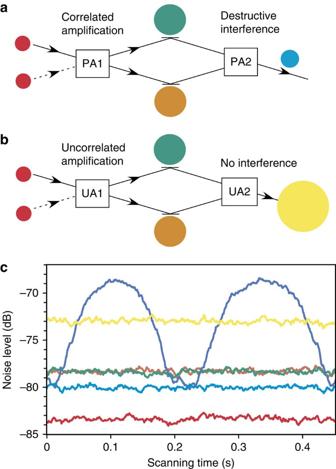Figure 2: The noise levels for the NCI. (a,b) Graphic representation for (a) correlated amplification (PA) with quantum interference or (b) uncorrelated amplification (UA) with no interference. Solid circles represent the noise with colours corresponding to the traces of the same colours in (c). The sizes of the circles correspond to the noise levels in (c) (not to scale). In (a), a coherent state at vacuum noise level (red) is input to the NCI together with the vacuum state at the unused input port (dashed line) and then amplified by PA1 (green and dark brown) but quantum destructive interference at PA2 brings the noise level back close to shot noise level (light blue). However in (b), without the interference, the noise level is further amplified by PA2 (yellow). (c) Measured noise levels at zero frequency span at the output: the dark blue trace is the noise level when the phaseφof the NCI is scanned; the yellow trace is the noise level when one arm of the NCI is blocked; the green and dark brown traces are the noise levels (noise gain) for individual amplifiers with vacuum input; the light blue trace is the noise level at dark fringe (φ=π) of the NCI; the red trace is the vacuum noise level, which is also the noise level for a CI at dark fringe. The centre frequency=1 MHz, frequency span=0, resolution bandwidth=100 kHz, video bandwidth=100 Hz. The scanning time is the time for phase scan via PZT voltage ramp and the scope running time. Figure 2: The noise levels for the NCI. ( a , b ) Graphic representation for ( a ) correlated amplification (PA) with quantum interference or ( b ) uncorrelated amplification (UA) with no interference. Solid circles represent the noise with colours corresponding to the traces of the same colours in ( c ). The sizes of the circles correspond to the noise levels in ( c ) (not to scale). In ( a ), a coherent state at vacuum noise level (red) is input to the NCI together with the vacuum state at the unused input port (dashed line) and then amplified by PA1 (green and dark brown) but quantum destructive interference at PA2 brings the noise level back close to shot noise level (light blue). However in ( b ), without the interference, the noise level is further amplified by PA2 (yellow). ( c ) Measured noise levels at zero frequency span at the output: the dark blue trace is the noise level when the phase φ of the NCI is scanned; the yellow trace is the noise level when one arm of the NCI is blocked; the green and dark brown traces are the noise levels (noise gain) for individual amplifiers with vacuum input; the light blue trace is the noise level at dark fringe ( φ = π ) of the NCI; the red trace is the vacuum noise level, which is also the noise level for a CI at dark fringe. The centre frequency=1 MHz, frequency span=0, resolution bandwidth=100 kHz, video bandwidth=100 Hz. The scanning time is the time for phase scan via PZT voltage ramp and the scope running time. Full size image The traces in light blue and red in Fig. 2c respectively show the measured noise levels at dark fringe setting for the NCI and the CI under the same condition when the fringes in Fig. 1c are measured. The observed noise level for the NCI is 3.3±0.3 dB higher than that of the CI. This is not what is predicted in previous paragraphs, that is, the noise level of the NCI is the same as that of the CI at the vacuum noise level. The higher measured output noise of the NCI is due to internal losses of the interferometer (more on this later). Even so, combined with the 7.4 dB of signal enhancement from Fig. 1c (it was shown in ref. 30 that the signal due to a small phase shift δ in HD of an interferometer has the same form as that in direct intensity detection), we still obtain an enhancement of 4.1±0.3 dB in signal-to-noise ratio for the NCI over the CI, that is, SNR NCI /SNR CI =4.1 dB=2.5. From equation (5), we know that the signal is proportional to δ 2 , whereas the noise measured in the experiment is the noise power. So, we have the phase measurement sensitivity as in rms value. As the CI has a phase measurement sensitivity at SNL [3] , our NCI beats the shot noise level by a factor of =1.6 in rms value. The simple theory in the previous part does not include losses in the system and predicts the continuous increase of the SNR with the gain of the amplifiers. Losses, however, will introduce extra vacuum noise, which is also amplified by PA1 and PA2 but is not correlated and cannot be cancelled, thus leading to higher noise level for the NCI than the CI but at a manageable level, as observed in Fig. 2c . The extra amplified vacuum noise will increase with the gain of the amplifiers in the same way as the phase signal. Therefore, this makes SNR independent of the gain at high gain [30] . This effect is shown in Fig. 3 where we plot in blue diamond shape the ratio of the output noise level of the interferometer at dark fringe (the light blue trace in Fig. 2c ) to the vacuum noise level (the red trace in Fig. 2c ) as a function of the average noise gain of individual amplifiers (the traces in green and dark brown in Fig. 2c ). Since the vacuum noise level is also the output noise level of the CI at dark fringe, this is also the noise level ratio of the NCI to the CI. Shown also in Fig. 3 in black square shape are the ratio of the signal level of the NCI to that of the CI, or the signal enhancement factor B S extracted from the fringes similar to Fig. 1c . Therefore, the ratio of the black square to the blue diamond gives the enhancement of the signal-to-noise ratio of the NCI over the CI, which is shown as red triangle in Fig. 3 . As seen in the figure, both the signal enhancement factor (black) and the noise level (blue) at the output increase with the amplifier gain in about the same rate at high gain. So, the signal-to-noise improvement factor (red) levels out at a gain of ~4 dB, in qualitative agreement with ref. 30 . 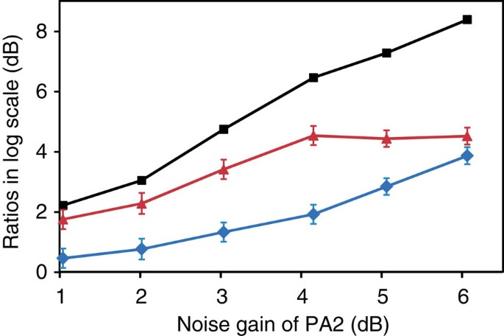Figure 3: Comparison between the NCI and the CI. The blue diamond-shaped data are for the ratio of the noise level of the idler output of the NCI to the vacuum noise level. The black squares are for the ratio of the signal level of the NCI to that of the CI or the signal enhancement factor. The red triangles are for the ratio of the SNR of NCI to that of the CI or the SNR enhancement factor. They are plotted as a function of the noise gain of PA2. The solid lines are for visual guidance. The SNR enhancement factor (red triangle) levels out at high gain because of the losses in the interferometer. The size of the error bars is one s.d., derived from the data of the traces similar to the light blue and red traces inFig. 2. Figure 3: Comparison between the NCI and the CI. The blue diamond-shaped data are for the ratio of the noise level of the idler output of the NCI to the vacuum noise level. The black squares are for the ratio of the signal level of the NCI to that of the CI or the signal enhancement factor. The red triangles are for the ratio of the SNR of NCI to that of the CI or the SNR enhancement factor. They are plotted as a function of the noise gain of PA2. The solid lines are for visual guidance. The SNR enhancement factor (red triangle) levels out at high gain because of the losses in the interferometer. The size of the error bars is one s.d., derived from the data of the traces similar to the light blue and red traces in Fig. 2 . Full size image Next, we characterize the effect of losses on the performance of the NCI by introducing some extra losses. First, we place an attenuator with loss L in front of the homodyne detector and vary the attenuation. 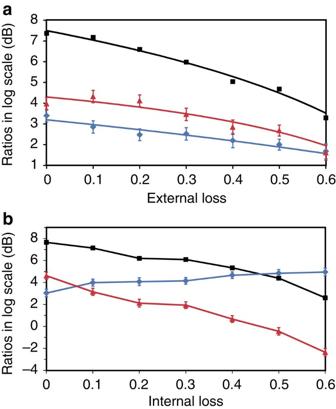Figure 4: Effect of losses on the enhancement of signal-to-noise ratio. (a) Extra external loss; (b) extra internal loss on the both arms. The blue diamond points are the output noise level above the vacuum level; the black square points are the signal enhancement factor; the red triangle points are the signal-to-noise ratio enhancement factor. Solid curves in (a) are from equation (7) withBS0=7.5 dB andN0=3.2 dB. The solid lines in (b) are for visual guidance. At small losses, the SNR enhancement factor (red triangle) is less sensitive to the external losses than to internal losses. The size of the error bars is one s.d., derived from the data of the traces similar to the light blue and red traces inFig. 2. Figure 4a shows the results. We can model the attenuator by a beam splitter of transmission 1− L . Then, the signal enhancement factor B S and noise N above vacuum noise level after the attenuator will change with the loss L by Figure 4: Effect of losses on the enhancement of signal-to-noise ratio. ( a ) Extra external loss; ( b ) extra internal loss on the both arms. The blue diamond points are the output noise level above the vacuum level; the black square points are the signal enhancement factor; the red triangle points are the signal-to-noise ratio enhancement factor. Solid curves in ( a ) are from equation (7) with B S0 =7.5 dB and N 0 =3.2 dB. The solid lines in ( b ) are for visual guidance. At small losses, the SNR enhancement factor (red triangle) is less sensitive to the external losses than to internal losses. The size of the error bars is one s.d., derived from the data of the traces similar to the light blue and red traces in Fig. 2 . Full size image where B S0 and N 0 are the respective values before the attenuator. So, the signal-to-noise ratio after the attenuator becomes The solid lines in Fig. 4a are fitted to equations (6) and (7) with B S0 =7.5 dB and N 0 =3.2 dB. So, the signal-to-noise improvement factor does not change much at small loss for large N 0 . This is well known for amplification process: the amplified noise is above the vacuum level so that the noise will decrease under loss just like the signal, making SNR less sensitive to external losses. This is quite different from the squeezed state scheme [5] , [6] in which the improvement will suffer under loss. For large loss, however, SNR will drop with the increase of the loss because the noise level is mostly vacuum noise already and won't decrease further. For the effect of internal loss, we place a variable attenuator in the paths of both arms of the NCI. We need to readjust the gain of PA2 to re-balance the interferometer so that it produces fringe visibility close to 100%. In the meantime, gain balancing also leads to optimized output noise levels shown Fig. 4b . As seen in Fig. 4b , the output noise level (blue diamond) increases as the loss increases—more uncorrelated vacuum noise enters the interferometer and gets amplified. However, the signal size (black square) drops for increased loss. Therefore, the improvement factor in signal-to-noise ratio decreases more quickly with internal loss ( Fig. 4b ) than with external loss ( Fig. 4a ). The effect of internal loss on the NCI is complicated so we cannot fit the data to a theoretical prediction. However, the general trend is correct qualitatively. We have demonstrated an SU(1,1) NCI with 4 dB improvement in signal-to-noise ratio in phase measurement over a CI operated under the same condition. The improvement is mostly limited by the loss inside the interferometer and is less sensitive to external loss than the squeezed state method. The improvement in signal-to-noise ratio comes from the increase in signal rather than the reduction of noise. Furthermore, if we inject squeezed states into the unused idler input port of PA1 (see Fig. 1a ), reduction of the noise of the interferometer is possible, leading to further improvement of signal-to-noise ratio. Therefore, the current scheme and the squeezed state scheme are complementary to each other. Notice that our NCI involves amplification of the input field whereas a conventional MZ interferometer (CI) does not. Therefore, it seems that the NCI uses more resources than the CI. However, according to refs 21 , 25 it is the photon number of the phase probing field that counts for the limit of sensitivity. Therefore, when we compare the performance of our NCI with the CI, we make sure that the light fields probing the phase change have the same intensity in both NCI and CI. When we reduce the intensity of the injected coherent state, this interferometer will approach to the originally proposed SU(1,1) interferometer by Yurke et al. [19] , which can have a phase measurement sensitivity reaching the Heisenberg limit. Our simple theoretical model shows that the sensitivity improvement increases with the gain. However, as we have shown in Fig. 3 , the internal loss of the interferometer is the main limiting factor in achieving higher sensitivity at higher gain. This is consistent with the results of ref. 30 and Demkowicz-Dobrzanski et al. [36] Then, it is natural to ask what kind of phase measurement sensitivity limit we can reach in our new interferometer. To answer that, we need to use Fisher information estimation method [37] . Unfortunately, our measurement technique, that is, the HD method, does not allow us to perform an analysis with Fisher information method, which requires photon counting technique. Phase estimate with Fisher information method for this new type of interferometer will be the topic in future researches. What we did in current work is to compare the performance of our new interferometer with a conventional MZ interferometer, which has the well-known SNL (1/ -dependence for phase measurement uncertainty), and show a 4-dB improvement in signal-to-noise ratio. The use of a nonlinear process to mix the signal and idler fields means that the two fields may have different frequencies. Indeed, in our experiment, the frequency difference between the signal and the idler fields is ~6 GHz. In fact, they may not necessarily be the same type of waves. This opens up a new way to construct hybrid interferometers involving different waves and thus broadens the scope of precision measurement involving interferometry. Detailed experimental arrangement The detailed experimental arrangement is shown in Fig. 5 . The two parametric amplifiers (PA1, PA2) employed for the NCI as shown in Fig. 1a are based on non-degenerate four-wave mixing process in two hot Rb-85 atomic vapour cells temperature-stabilized at 117 °C (ref. 29 ); see inset of Fig. 5 for energy diagram of relevant components). They are respectively pumped by a vertically polarized beam (P1, P3) at a maximum power of 400 mW with a waist of 500 μm. The pump beams are from a Ti:sapphire laser frequency-stabilized to a stable reference cavity. The pump beams are detuned about 0.8 GHz above the transition line of Rb-85 F =2→ F ′ at 795 nm. The pump power can be adjusted with a combination of polarization beam splitters (PBS) and half-wave plates. A horizontally polarized seed beam (also known as ‘signal’) with waist of 200 μm is injected with an angle of 0.4° relative to the pump. The ‘signal’ beam is 3.04 GHz red shifted from the pump beam by an acousto-optic modulator in double-pass configuration. The pump and signal beams are combined with a Glan-laser PBS before being sent into the atomic cell. At the output of the atomic cell, the seed signal beam is amplified with a gain that depends on the power and frequency detuning of the pump beam. The amplification of the signal beam is accompanied by a conjugate beam (called ‘idler’) with a frequency of 3.04 GHz blue shift from the pump at the other side of the pump beam. The second cell is identical to the first one except that both the signal and the idler fields have inputs that are from the first cell. A 4-F imaging system (L1, L2) is used to mode match the fields of the two cells. 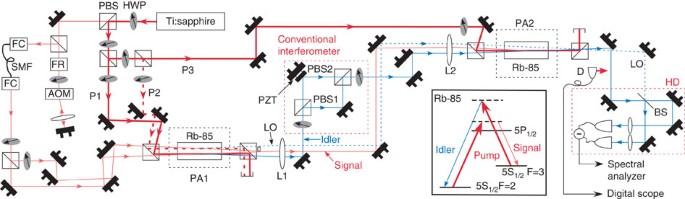Figure 5: Detailed experimental arrangement. An NCI is formed with PA1 and PA2 with injection at PA1. PBS, polarization beam splitter; HWP, half-wave plate; FR, Faraday rotator; AOM, acousto-optic modulator; FC, fibre coupler; SMF, single mode fibre; P1, P2, P3, pumps for four-wave mixing (4WM); PA1, PA2, 4WM-parametric amplifiers; L1, L2, lenses for 4F-imaging system; PZT, piezo-electric transducers; LO, local oscillator for HD; HD, homodyne detection; D, detector. A conventional MZ interferometer (CI) is formed by flipping in PBS1 and PBS2 on flipping mounts together with corresponding HWPs for minimum change to the optical pathes. Inset: Rb-85 atomic energy level diagram for four-wave mixing. Phase change is introduced through PZT for both the NCI and the CI. Figure 5: Detailed experimental arrangement. An NCI is formed with PA1 and PA2 with injection at PA1. PBS, polarization beam splitter; HWP, half-wave plate; FR, Faraday rotator; AOM, acousto-optic modulator; FC, fibre coupler; SMF, single mode fibre; P1, P2, P3, pumps for four-wave mixing (4WM); PA1, PA2, 4WM-parametric amplifiers; L1, L2, lenses for 4F-imaging system; PZT, piezo-electric transducers; LO, local oscillator for HD; HD, homodyne detection; D, detector. A conventional MZ interferometer (CI) is formed by flipping in PBS1 and PBS2 on flipping mounts together with corresponding HWPs for minimum change to the optical pathes. Inset: Rb-85 atomic energy level diagram for four-wave mixing. Phase change is introduced through PZT for both the NCI and the CI. Full size image A CI of MZ type is formed in the path of the idler field with a pair of flipping PBS (PBS1, PBS2) and a beam-redirecting mirror. In this way, minimum alignment is required to switch between CI and NCI. We block the signal arm and the pump to cell 2 (P3) when we operate the CI. A PZT-mounted mirror (PZT) is placed in both interferometers as the phase modulator so that we can compare the performance of both interferometers under the same phase change. Since the PBS splits the idler beam into two equal parts in the CI and reduces the phase-sensing intensity to half, we need to increase the injected signal at cell 1 to bring the phase-sensing intensity of the CI to the same level as that of the NCI ( I ps =60 μW with I seed =16 μW). A regular silicon photo-detector (D) is placed in the idler output port of the NCI, which is also the output port for the CI. This detector records the fringes of the NCI and the CI in a digital scope, as shown in Fig. 1c . The noise performance of the NCI is measured by HD (with a 98% homodyne efficiency) at the output of the idler side of the NCI under different circumstances. The local oscillator of 726 μW for HD is obtained from cell 1 with another seed (196 μW) and pump (P2=300 mW) [34] . The local oscillator goes through the same imaging system to match its mode with those in the interferometer. The shot noise level is ~10 dB above the electronic noise level. How to cite this article: Hudelist, F. et al. Quantum metrology with parametric amplifier-based photon correlation interferometers. Nat. Commun. 5:3049 doi: 10.1038/ncomms4049 (2014).